Total synthesis and antimicrobial evaluation of natural albomycins against clinical pathogens Development of effective antimicrobial agents continues to be a great challenge, particularly due to the increasing resistance of superbugs and frequent hospital breakouts. There is an urgent need for more potent and safer antibiotics with novel scaffolds. As historically many commercial drugs were derived from natural products, discovery of antimicrobial agents from complex natural product structures still holds a great promise. Herein, we report the total synthesis of natural albomycins δ 1 ( 1a ), δ 2 ( 1b ), and ε ( 1c ), which validates the structures of these peptidylnucleoside compounds and allows for synthetic access to bioactive albomycin analogs. The efficient synthesis of albomycins enables extensive evaluations of these natural products against model bacteria and clinical pathogens. Albomycin δ 2 has the potential to be developed into an antibacterial drug to treat Streptococcus pneumoniae and Staphylococcus aureus infections. Sideromycins are a class of antibiotics covalently linked to siderophores [1] . They are actively transported into bacterial cells via siderophore uptake pathways commonly found in bacterial pathogens, by the so-called “Trojan horse” strategy, resulting in outstanding cell envelope permeability and very low minimum inhibitory concentrations (MICs). These pathogen-specific antibiotics are promising drug candidates for the treatment of various bacterial infections [2] , [3] , [4] . A few naturally occurring sideromycins have been discovered. Among these, albomycins, originally reported as grisein, were first isolated from soil microorganism Streptomyces griseus in 1947 [5] , [6] , [7] , [8] , [9] . Albomycins exhibited potent inhibitory activities against a number of Gram-negative, as well as Gram-positive bacteria, including multi-drug resistant strains [1] , [10] , [11] . For instance, albomycins exhibited an MIC value of 10 ng/mL against Streptococcus pneumoniae and 5 ng/mL against Escherichia coli , which is almost tenfold more potent than penicillin [12] . Moreover, no toxicity was observed during in vivo studies of albomycins, and it was well tolerated and safe up to a maximum dose evaluated in mice [10] . Albomycins have been successfully used to treat human bacterial infections in the Soviet Union [10] . The structures of albomycins were fully elucidated by Benz and coworkers in 1982 [13] , [14] , 35 years after their initial isolation. Albomycins δ 1 ( 1a ), δ 2 ( 1b ), and ε ( 1c ) are all composed of a tri-δ- N -hydroxy-L-ornithine peptide siderophore and a thionucleoside warhead with six consecutive chiral centers, and differ only in the C4 substituent (R) of the pyrimidine nucleobase (Fig. 1 ). As for 1b , the thionucleoside warhead is a potent seryl-tRNA synthetase inhibitor known as SB-217452 [15] . The highly complex and densely functionalized structures, together with their important therapeutic potential, have made albomycins attractive targets for synthesis. Different synthetic strategies for the tri-δ- N -hydroxy-L-ornithine peptide siderophore have been described by the groups of Benz [16] , [17] and Miller [18] , [19] , [20] . The synthesis of the thionucleoside moiety of 1a was briefly described by Holzapfel et al. in 1991 [21] , though with incomplete data. However, no total synthesis of albomycins has been reported. In one study [22] , an oxygen analog of 1a was synthesized. Surprisingly, a single replacement of the sulfur with oxygen resulted in the complete loss of antibacterial activity, suggesting a critical role of the sulfur atom in the activity of albomycins. A biosynthetic approach has also been attempted for the generation of albomycin analogs [23] , but albomycin production by S. griseus is difficult and has yet to be scaled up efficiently [24] . Herein, we describe the total synthesis of the three natural albomycins ( 1a – c ), which features a Pummerer reaction for nucleobase introduction and an aldol reaction to expand the side chain of thionucleoside. Their biological evaluations demonstrate that albomycin δ 2 is a promising lead candidate for treating S. pneumoniae and S . aureus infections and warrants further development. Fig. 1 Chemical structures of albomycins δ 1 , δ 2 , and ε , and their synthetic strategies. The key disconnections involve a Pummerer reaction for nucleobase introduction and an aldol reaction to expand the side chain of thionucleoside. tBu tert -butyl, Bz benzoyl, Fmoc fluorenylmethyloxycarbonyl, PMB p -methoxybenzyl Full size image Synthetic strategy The retrosynthetic analysis of albomycins ( 1a – c ) in a collective fashion is shown in Fig. 1 . The amide bond linking to the thionucleoside core was first disconnected to generate tetrapeptide fragment 2 and thionucleosides 3a – c . Tetrapeptide 2 could be readily accessed via the condensations of tripeptide 4 with L-serine tert -butyl ester. Tripeptide 4 could be derived from amino acid 6 , which could arise from the direct oxidation of protected L-ornithine 8 . We anticipated that thionucleosides 3a – c could be installed by substrate-directed asymmetric aldol condensation reaction from thionucleosides 5a - c , which could in turn be prepared through a Pummerer reaction from thiosugar 7 and uracil. Thiosugar 7 could be further traced back to the known L-(+)-lyxose derivative 9 . Due to the structural feature and labile nature of albomycins, the protecting group strategy had to be delicately selected to accomplish the total synthesis. Because of the presence of reducible hydroxamic acids in the siderophore moiety and an imine group in the thionucleoside moiety of 1b and 1c , protecting groups such as Cbz and Bn which usually need to be deprotected under reducing conditions of H 2 and Pd/C in the final stage were avoided. As for the hydroxyl groups in the thionucleoside fragment, orthogonality of protecting groups and their influence on stereoselectivity of uracilation were also key considerations. Total synthesis of albomycins δ 1 , δ 2 , and ε Our synthetic efforts commenced with the preparation of tetrapeptide 2 (Fig. 2 ). The core component hydroxamic acid 6 of tetrapeptide 2 was first synthesized from N 2 -Boc-L-ornithine tert -butyl ester 8 [25] . Oxidation of the free amine in N 2 -Boc-L-ornithine tert -butyl ester 8 with benzoyl peroxide [25] , [26] , [27] , followed by acylation under biphasic conditions afforded the fully protected hydroxamate 6 in 80% yield. Removal of tert -butyl-carbonate (Boc) and tert -butyl ( t -Bu) groups with trifluoroacetic acid (TFA) provided the TFA salt 10 . The resulting amine group was protected with Fmoc to deliver acid 11 in 91% yield over two steps. Then, we turned to coupling 11 and 10 under active ester-mediated coupling conditions (DCC, NHS) [20] , which proceeded smoothly to produce dipeptide 12 . Unfortunately, application of the same conditions to synthesize tripeptide 4 led to significant epimerization. Failure to optimize the condition after numerous efforts prompted us to explore an alternative strategy. Fortunately, under active amide-mediated coupling conditions developed by Katritzky [28] , [29] , [30] , [31] , tripeptide 4 could be obtained in an iterative fashion from 11 in 77% yield over two steps without any detectable epimerization. Tripeptide 4 was condensed with L-serine tert -butyl ester hydrochloride in the presence of HATU and DIPEA to generate tert -butyl ester 13 in 95% yield. Treatment of 13 with TFA in dichloromethane at 0 °C proceeded smoothly to yield the corresponding tetrapeptide 2 . Fig. 2 Synthesis of tetrapeptide 2 . Reagents and conditions: a BPO (2.0 equiv), pH 10.5 buffer, CH 2 Cl 2 , 3 h, then AcCl (1.2 equiv), CH 2 Cl 2 , 80%; b TFA, H 2 O, 12 h; c Fmoc-OSu (1.2 equiv), Et 3 N (3.0 equiv), DMF, −15 °C, overnight, 91% (2 steps); d BtH (4.0 equiv), SOCl 2 (1.0 equiv), THF, 50 min, then 10 (1.1 equiv), Et 3 N (3.1 equiv), CH 3 CN/H 2 O (5:2), −15 °C, 2 h, 12 : 89%, 4 : 87%; e H-Ser( t Bu)-O t Bu hydrochloride (1.1 equiv), HATU (1.5 equiv), DIPEA (2.0 equiv), DMF, −15 °C, 2 h, 95%; f TFA, H 2 O, CH 2 Cl 2 , 0 °C, 18 h. BPO benzoyl peroxide, AcCl acetyl chloride, TFA trifluoroacetic acid, Fmoc-OSu N -(9-fluorenylmethoxycarbonyloxy)-succinimide, DMF N , N -dimethyformamide, DCC dicyclohexylcarbodiimide, NHS N -hydroxysuccinimide, BtH 1 H -benzotriazole, THF tetrahydrofuran, HATU 1-[bis(dimethylamino) methylene]-1H-1,2,3-triazolo [4,5-b] pyridinium 3-oxid hexafluorophosphate, DIPEA N , N -diisopropylethylamine Full size image With tetrapeptide 2 in hand, we initiated the synthesis of thionucleosides 5a - c (Fig. 3 ). At first, lactone 9 [32] was transformed into lactone 14 by a two-step sequence involving Mitsunobu reaction and removal of the isopropylidene protecting group with TFA. Selective mono-tosylation of lactone 14 with tosyl chloride/DABCO generated tosylate 15 in 87% yield. In this case, use of pyridine led to low conversion because of its weaker basicity, whereas Et 3 N to a bis-tosylation byproduct which further underwent elimination to produce the corresponding α,β -unsaturated tosylate. The transformation of 15 to 16 with K 2 CO 3 in MeOH at room temperature gave the product with the undesired configuration at C4' exclusively. A variety of bases and temperatures were examined for the 5-membered thio-ring closure reaction, and eventually the use of K 2 CO 3 as a base at −30 °C in MeOH smoothly led to 16 in 81% yield without any detectable epimerization. It was surprising that the reaction temperature had such an impact on the stereoselectivity. As mentioned above, the proper choice of protecting group for the trans -1,2-diol is crucial, because the neighboring group effect could influence the stereoselectivity of the following uracilation reaction [33] . Initially, when the trans -1,2-diol was protected as a diester, the Pummerer reaction indeed provided the desired product as a single diastereomer with moderate yield. However, this protected diester was incompatible with the subsequent selective methyl ester reduction and later stage aldol reaction. Thus, trans -1,2-diol 15 was protected with 2,3-butanedione under acid catalysis, followed by reduction of the methyl ester with DIBAL-H to afford sulfide 7 . Treatment of sulfide 7 with m -CPBA provided the corresponding sulfoxide 17 in 95% yield, and subsequent Pummerer reaction [34] , [35] with DIPEA as a base gave rise to 18 and epi - 18 in 86% yield as a 1:1 diastereoisomeric mixture. Commonly used Et 3 N was not suitable for the Pummerer reaction because it could act as a nucleophile, leading to formation of a triethylammonium adduct, and thus reduced yield [36] . The N -methyl group was introduced by a conventional procedure to afford 5a , which is an advanced intermediate for the synthesis of albomycin δ 1 . The structure of 5a was verified by X-ray crystallographic analysis (Fig. 3 ). To achieve the synthesis of albomycin δ 2 and ε , a practical access to the imine 20 was required. First, 18 was protected as its TBS ether 19 , which was treated with TPSCl in the presence of DMAP and Et 3 N, followed by NH 4 OH to produce a cytosine derivative in 90% yield over two steps in one pot, and then methylation of N3 delivered 20 in 96% yield. For the subsequent installation of the N4 carbamoyl group, aminolysis of N 4-phenoxycarbonyl [37] did not take place due to the steric hindrance of the N3 methyl group. Inspired by the N -PMB carbamoylimidazole urea formation reported by Batey et al. [38] , we developed a scalable and efficient protocol to prepare 22b . In the presence of Et 3 N, 20 was allowed to react with 21 under reflux, giving rise to 22b in 96% yield. Additionally, Fmoc was chosen as the protecting group for 20 , leading to 22c , which is a key intermediate for the synthesis of albomycin ε. Fig. 3 Synthesis of intermediates 5a - c and X-ray crystal-structure diagram of 5a . Reagents and conditions: a AcSH (2.2 equiv), DIAD (2.2 equiv), PPh 3 (2.2 equiv), THF, 0 °C, 5 h, 89%; b TFA, CH 2 Cl 2 , H 2 O, 5 h, 90%; c TsCl (1.2 equiv), DABCO (1.1 equiv), CH 3 CN, 1 h, 87%; d K 2 CO 3 (1.5 equiv), MeOH, −30 °C, 3 h, 81%; e 2,3-butanedione (1.2 equiv), trimethoxymethane (4.0 equiv), CSA (0.1 equiv), MeOH, reflux, 24 h, 86%; f DIBAL-H (2.1 equiv), CH 2 Cl 2 , 0 °C, 2 h, 98%; g m -CPBA (1.0 equiv), CH 2 Cl 2 , 0 °C, 0.5 h, 95%; h uracil (2.0 equiv), TMSOTf (8.0 equiv), DIPEA (8.0 equiv), toluene, CH 2 Cl 2 , 3 h, d.r. 1:1, 86%; i methyl iodide (1.2 equiv), K 2 CO 3 (1.5 equiv), DMF, 2 h, 98%; j TBSCl (2.2 equiv), imidazole (2.2 equiv), DMAP (0.1 equiv), CH 3 CN, 2 h, 98%; k TPSCl (2.0 equiv), Et 3 N (2.0 equiv), DMAP (2.0 equiv), CH 3 CN, 1 h, then NH 4 OH, 20 h, 90%; l methyl iodide (3.0 equiv), DMAc, 3.5 h, 96%; m 21 (2.0 equiv), Et 3 N (1.0 equiv), THF, reflux, 96%. n Fmoc-Cl (2.0 equiv), NaHCO 3 (4.0 equiv), THF/H 2 O, 90%; o TBAF (1.3 equiv), THF, 2 h, 95%; p HF·pyridine (5.0 equiv), THF, 36 h, 95%. AcSH thiolacetic acid, DIAD diisopropyl azodiformate, DABCO 1,4-diazabicyclo[2.2.2]octane, CSA camphorsulfonic acid, DIBAL-H diisobutylaluminum hydride, TPSCl 2,4,6-triisopropylbenzenesulfonyl chloride, DMAP 4-dimethylaminopyridine, DMAc N , N -dimethylacetamide, TBAF tetrabutylammonium fluoride Full size image With fragments 5a – c in hand, the next challenge was to install the side chain with the desired stereochemistry (Fig. 4 ). Oxidation of alcohols 5a – c with IBX gave the corresponding aldehydes 23a – c in excellent yields. Side-chain extension via aldol reaction required a delicate choice of protecting groups for the glycine moiety, which is essential for good stereoselectivity. Inspired by Trost’s work [39] , we found that the lithium salt of N -(diphenylmethylene) glycine methyl ester could react with aldehydes 23a – c at −78 °C, and subsequent treatment of the condensation products with 2 M aqueous HCl yielded 3a (86%, 2 steps, d.r. 4:1), 3b (83%, 2 steps, d.r. 3:1), and 3c (75%, 2 steps, d.r. 3:1) respectively. The structures of 3a and 3b were unambiguously established by X-ray crystallographic analysis, and the molecular structure of 3c was substantiated by X-ray crystallography of its benzoyl derivative 3c' (Fig. 4 ). Fig. 4 Synthesis of fragments 3a – c and X-ray crystal-structure diagrams of 3a , 3b , and 3c' . Reagents and conditions: a IBX (2.0 equiv), CH 3 CN, 55 °C, 5 h; b 24 (1.1 equiv), LDA (1.1 equiv), THF, −78 °C, then 2 M HCl, 3a : 86% (d.r. 4:1), 3b : 83% (d.r. 3:1), 3c : 75% (d.r. 3:1), (over 2 steps). IBX 2-iodoxybenzoic acid, LDA lithium diisopropylamide Full size image With key fragments 2 and 3a – c in place, their assembly into albomycins ( 1a – c ) was embarked (Fig. 5 ). Thionucleosides 3a – c were first condensed with tetrapeptide 2 to afford 25a – c in excellent yields. The final deprotection steps from 25a – c to the final albomycins ( 1a – c ) required delicate adjustments of the reaction conditions in order to preserve the sensitive amide bond [40] on the cytosine of 1b and 1c . First, oxidative deprotection of the N -PMB group in 25b proceeded smoothly. Addition of CF 3 CO 2 H and H 2 O to the resulting crude product removed the bisacetal moiety within the molecules. The reaction time for these two deprotection steps needed to be carefully controlled, otherwise it would lead to hydrolysis of the imine. After surveying numerous reaction conditions, we found that aqueous K 2 CO 3 (150 mg/mL) could efficiently remove the remaining protecting benzoyl, methyl ester, and Fmoc groups in one pot to afford albomcyin δ 2 ( 1b ). These three deprotection steps ( 25b to 1b ) were carried out without purifying the intermediates and the final product albomycin δ 2 ( 1b ) was purified with Sephadex TM G-15. We subsequently exploited the flexibility of this sequential deprotection. To our pleasure, following the same protocals, both albomycins δ 1 ( 1a ) and ε ( 1c ) were obtained in good yields. It’s worth noting that albomcyin ε ( 1c ) was not stable in D 2 O, and slowly converted to albomycin δ 1 ( 1a ) over time. Albomycin δ 2 ( 1b ) was much more stable than albomcyin ε ( 1c ), and remained unchanged in D 2 O at 4 °C for over one month. Fig. 5 Total synthesis of albomycins δ 1 , δ 2 , and ε . Reagents and conditions: a HATU (1.5 equiv), DIPEA (2.0 equiv), DMF, −15 °C, 2 h, 25a : 93%, 25b : 91%, 25c : 90%; b CAN (10.0 equiv), CH 3 CN/H 2 O, 30 min; c TFA, H 2 O, 1 h; d K 2 CO 3 , MeOH, H 2 O, 1a : 80% (over 2 steps), 1b : 72% (over 3 steps), 1c : 75% (over 2 steps). CAN ceric ammonium nitrate Full size image Biological assessment As the three naturally occurring albomycins became synthetically accessible, we evaluated their potential as therapeutic agents and determined their MIC values against three Gram-positive and three Gram-negative bacteria species following the protocol from the Clinical and Laboratory Standards Institute (CLSI). Commercial antibiotic, ciprofloxacin, was used as a positive control in the MIC determination experiment. 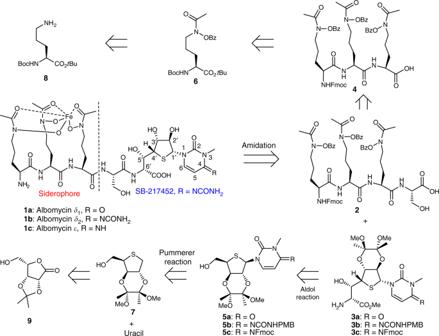Fig. 1 Chemical structures of albomycinsδ1,δ2, andε, and their synthetic strategies. The key disconnections involve a Pummerer reaction for nucleobase introduction and an aldol reaction to expand the side chain of thionucleoside.tButert-butyl,Bzbenzoyl,Fmocfluorenylmethyloxycarbonyl,PMBp-methoxybenzyl As shown in Table 1 , albomycin δ 1 ( 1a ) and δ 2 ( 1b ) exhibited 8-fold more potency than ciprofloxacin against S. pneumoniae ATCC 49619. 1b inhibited S. aureus USA 300 strain NRS384 [41] , a virulent methicillin resistant MRSA strain, with an MIC of 0.125 µg/mL, and was 16-fold more potent than ciprofloxacin. 1b exhibited an MIC value of 0.5 µg/mL against Bacillus subtilis ATCC 6633, which was less active compared to ciprofloxacin. As for Escherichia coli BJ 5183 [42] , 1b showed about 8-fold higher potency than 1a . Particularly impressive is the potency of compound 1a towards the fastidious Neisseria gonorrhoeae ATCC 49226 with a 3.9 ng/mL MIC value while 1b was completely inactive. These results led us to conclude that the C4 substituent of nucleobase in albomycins played an important role rendering their antibacterial activity. Biochemical analysis of albomycin nucleobase analogs will test this hypothesis. All three albomycins displayed no activity towards Gram-negative bacteria Salmonella typhi , and albomycin ε ( 1c ) was inactive to all these strains, which was previously unknown. Table 1 MIC values (μg/mL) of albomycins δ 1 ( 1a ), δ 2 ( 1b ), and ε ( 1c ) Full size table World Health Organization (WHO) published a priority list of antibiotic-resistant pathogenic bacteria for developing new and effective antibiotic treatments. Both S. pneumoniae and S. aureus are on the list due to their increasing multidrug resistance. Ciprofloxacin, vancomycin and penicillin G are on the WHO Model List of Essential Medicines (EML). Penicillin G is among the first medications against bacterial infections and vancomycin has been hailed as the last line of defense. 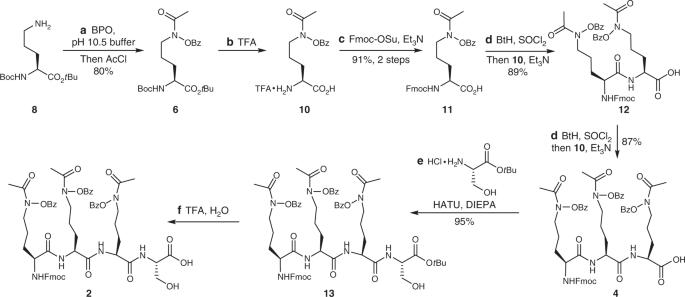Fig. 2 Synthesis of tetrapeptide2. Reagents and conditions:aBPO (2.0 equiv), pH 10.5 buffer, CH2Cl2, 3 h, then AcCl (1.2 equiv), CH2Cl2, 80%;bTFA, H2O, 12 h;cFmoc-OSu (1.2 equiv), Et3N (3.0 equiv), DMF, −15 °C, overnight, 91% (2 steps);dBtH (4.0 equiv), SOCl2(1.0 equiv), THF, 50 min, then10(1.1 equiv), Et3N (3.1 equiv), CH3CN/H2O (5:2), −15 °C, 2 h,12: 89%,4: 87%;eH-Ser(tBu)-OtBu hydrochloride (1.1 equiv), HATU (1.5 equiv), DIPEA (2.0 equiv), DMF, −15 °C, 2 h, 95%;fTFA, H2O, CH2Cl2, 0 °C, 18 h.BPObenzoyl peroxide,AcClacetyl chloride,TFAtrifluoroacetic acid,Fmoc-OSuN-(9-fluorenylmethoxycarbonyloxy)-succinimide,DMFN,N-dimethyformamide,DCCdicyclohexylcarbodiimide,NHSN-hydroxysuccinimide,BtH1H-benzotriazole,THFtetrahydrofuran,HATU1-[bis(dimethylamino) methylene]-1H-1,2,3-triazolo [4,5-b] pyridinium 3-oxid hexafluorophosphate,DIPEAN,N-diisopropylethylamine To explore the potential to develop albomycin δ 2 into an effective antibiotic, we screened albomycin δ 2 against a random collection of 27 clinical S. pneumoniae and S. aureus isolates (three of them are MRSA strains), and compared it with ciprofloxacin, vancomycin, and penicillin G (Table 2 ) in inhibiting the growth of these clinical pathogens. All these S. pneumoniae and S. aureus strains were freshly isolated from patients in clinic. As shown in Table 2 , albomycin δ 2 exhibited excellent anti- S. pneumoniae and S. aureus activities better than the other three antibiotics in most cases, while many of these strains displayed severely natural resistance to penicillin G. The MIC values of albomycin δ 2 were well below those of ciprofloxacin, vancomycin, and penicillin G, and in a number of cases reaching 1000 times lower. 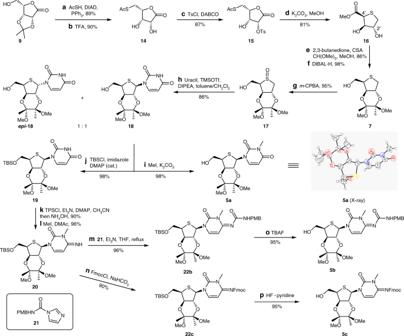Fig. 3 Synthesis of intermediates5a-cand X-ray crystal-structure diagram of5a. Reagents and conditions:aAcSH (2.2 equiv), DIAD (2.2 equiv), PPh3(2.2 equiv), THF, 0 °C, 5 h, 89%;bTFA, CH2Cl2, H2O, 5 h, 90%;cTsCl (1.2 equiv), DABCO (1.1 equiv), CH3CN, 1 h, 87%;dK2CO3(1.5 equiv), MeOH, −30 °C, 3 h, 81%;e2,3-butanedione (1.2 equiv), trimethoxymethane (4.0 equiv), CSA (0.1 equiv), MeOH, reflux, 24 h, 86%;fDIBAL-H (2.1 equiv), CH2Cl2, 0 °C, 2 h, 98%;gm-CPBA (1.0 equiv), CH2Cl2, 0 °C, 0.5 h, 95%;huracil (2.0 equiv), TMSOTf (8.0 equiv), DIPEA (8.0 equiv), toluene, CH2Cl2, 3 h, d.r. 1:1, 86%;imethyl iodide (1.2 equiv), K2CO3(1.5 equiv), DMF, 2 h, 98%;jTBSCl (2.2 equiv), imidazole (2.2 equiv), DMAP (0.1 equiv), CH3CN, 2 h, 98%;kTPSCl (2.0 equiv), Et3N (2.0 equiv), DMAP (2.0 equiv), CH3CN, 1 h, then NH4OH, 20 h, 90%;lmethyl iodide (3.0 equiv), DMAc, 3.5 h, 96%;m21(2.0 equiv), Et3N (1.0 equiv), THF, reflux, 96%.nFmoc-Cl (2.0 equiv), NaHCO3(4.0 equiv), THF/H2O, 90%;oTBAF (1.3 equiv), THF, 2 h, 95%;pHF·pyridine (5.0 equiv), THF, 36 h, 95%.AcSHthiolacetic acid,DIADdiisopropyl azodiformate,DABCO1,4-diazabicyclo[2.2.2]octane,CSAcamphorsulfonic acid,DIBAL-Hdiisobutylaluminum hydride,TPSCl2,4,6-triisopropylbenzenesulfonyl chloride,DMAP4-dimethylaminopyridine,DMAcN,N-dimethylacetamide,TBAFtetrabutylammonium fluoride The influence of iron concentration on the antibacterial activity was also studied by conducting assays in iron-rich and iron-deficient media (Table 3 ). The antibiotic activity of albomycin δ 2 against S . pneumoniae strains was significantly increased in iron-deficient media, which most closely mimics the physiological situation in a human host, wherein iron is sequestered in macromolecules such as heme [43] . Two isolates, strains S15 and S29, which showed the most resistance to albomycin δ 2 in iron-rich media, became highly susceptible under iron-depleted conditions. The MIC values of albomycin δ 2 against S . aureus and E . coli strains were not influenced by iron concentration. The three control antibiotics did not show any dependence on iron concentration in any of the strains tested. These results suggest that albomycin δ 2 is a promising antibiotic candidate for further clinical drug development. Table 2 MIC values (µg/mL) of albomycin δ 2 ( 1b ) against clinical isolates of S. pneumoniae and S. aureus Full size table Table 3 MIC values (μg/mL) of albomycin δ 2 ( 1b ) against S. pneumoniae, S. aureus and E. coli strains in MHII and MHII-Fe Full size table In summary, the successful execution of the convergent strategy has led to the total synthesis of albomycins δ 1 ( 1a ), δ 2 ( 1b ), and ε ( 1c ). Antibacterial assessment of albomycins revealed that C4 substituent on the nucleobase in albomycin plays an essential role in their antibacterial activity. Albomycin δ 2 exhibited potent antimicrobial activities against clinical S. pneumoniae and S. aureus isolates including MRSA. Further studies to evaluate albomycin δ 2 as a potentially effective and safe antibiotic are ongoing. General All air-sensitive and water-sensitive reactions were carried out under a nitrogen atmosphere with dry solvents under anhydrous conditions, unless otherwise noted. Tetrahydrofuran (THF) was distilled over sodium and benzophenone, dichloromethane (CH 2 Cl 2 ), N , N -dimethylformamide (DMF), triethylamine (Et 3 N), and N , N -diisopropylamine (DIPEA) over calcium hydride. All other solvents, as well as starting materials and reagents were obtained from commercial sources and used without further purification. Reactions were monitored by analytical thin-layer chromatography (TLC) on Merck silica gel 60 F 254 plates (0.25 mm), visualized by ultraviolet light and/or by staining with phosphomolybdic acid in EtOH. Retention factor (R f ) values were measured using a 5 × 2 cm TLC plate in a developing chamber containing the solvent system described. Yields refer to the isolated yields after silica gel flash column chromatography, unless otherwise stated. 1 H NMR spectra were obtained on an Agilent 400MR or 600MR DD2 spectrometer at ambient temperature. Chemical shifts were reported in parts per million (ppm), relative to either a tetramethylsilane (TMS) internal standard or the signals due to the solvent. 13 C NMR spectra were obtained with proton decoupling on an Agilent 400MR or 600MR DD2 (100 MHz or 150 MHz) spectrometer and were reported in ppm with residual portium for internal standard. Multiplicity is defined as: s = singlet; d = doublet; t = triplet; q = quartet; m = multiplet, br = broad, or combinations of the above. Coupling constants (J) are reported in Hertz. High resolution mass spectra were obtained on a Bruker SolariX 7.0 T spectrometer. Melting point was determined by WRS-2A Digital Melting Point Apparatus. Optical rotations were measured with a Rudolph polarimeter. Crystallographic data were obtained from a single-crystal X-ray diffractometer. Further experimental data For NMR spectra of the synthesized compounds, see Supplementary Figs. 1–62 . For detailed experimental procedures, see Supplementary Figs. 63–92 , and Supplementary Methods. For the comparisons of 1 H and 13 C NMR spectroscopic data of the natural and synthetic albomycin δ 2 , see Supplementary Tables 1 and 2 . For the crystallographic data of compounds 3a , 3b , 3c ' , and 5a , see Supplementary Figs. 93–96 , and Supplementary Tables 3–6 . Clinical pathogens isolation and identification The clinical pathogens were isolated according to National Guide to Clinical Laboratory Procedures and characterized by culturing in the specifically appropriate media followed by the VITEK mass spectrometry microbial identification system (bioMerieux, France). Antimicrobial susceptibility was performed for all tested clinical bacterial strains by 96-well microdilution method following Clinical and Laboratory Standards Institute (CLSI) recommendations. 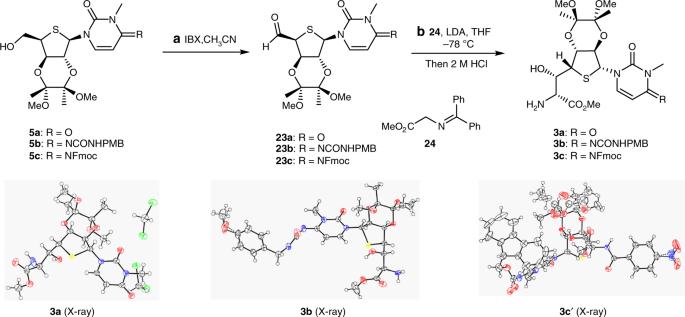Fig. 4 Synthesis of fragments3a–cand X-ray crystal-structure diagrams of3a,3b, and3c'. Reagents and conditions:aIBX (2.0 equiv), CH3CN, 55 °C, 5 h;b24(1.1 equiv), LDA (1.1 equiv), THF, −78 °C, then 2 M HCl,3a: 86% (d.r. 4:1),3b: 83% (d.r. 3:1),3c: 75% (d.r. 3:1), (over 2 steps).IBX2-iodoxybenzoic acid,LDAlithium diisopropylamide 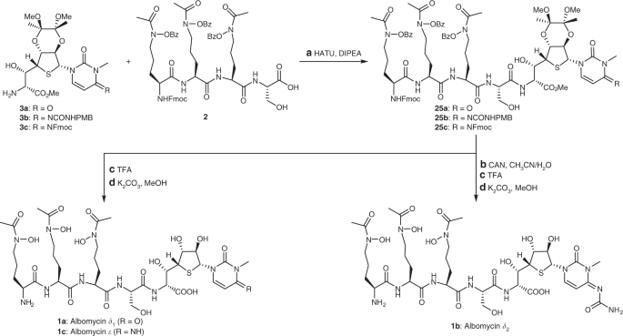Fig. 5 Total synthesis of albomycinsδ1,δ2, andε. Reagents and conditions:aHATU (1.5 equiv), DIPEA (2.0 equiv), DMF, −15 °C, 2 h,25a: 93%,25b: 91%,25c: 90%;bCAN (10.0 equiv), CH3CN/H2O, 30 min;cTFA, H2O, 1 h;dK2CO3, MeOH, H2O,1a: 80% (over 2 steps),1b: 72% (over 3 steps),1c: 75% (over 2 steps).CANceric ammonium nitrate Susceptibility testing Minimal inhibitory concentration (MIC) assays were adapted according to the recommendations of the Clinical and Laboratory Standard Institute (CLSIM07). For N. gonorrhoeae , MICs were determined by the standard agar dilution method on GC medium base with Isovitalex (Topbio, Shandong, China) at 37 °C with 5% CO 2 ; for S. pneumoniae , MICs were tested using 96-well microdilution plates in Mueller–Hinton broth II with 5% horse-blood (Solarbio, Beijing, China) at 37 °C with 5% CO 2 ; other strains were detected by the standard 96-well microdilution method in Mueller–Hinton broth II (Solarbio, Beijing, China) at 37 °C. Dilutions of the compound were made in quadruplicate in 96-well culture dishes. Strains were taken from an exponentially growing culture and diluted to 5 × 10 5 CFU/mL. The bacteria were cultured in the presence of tested compounds for about 20 h and bacterial growth was monitored visually following the CLSI guidelines. S. aureus ATCC 29213, S. pneumoniae ATCC 49619, and E.coli ATCC 25922 were used as quality control strains, which were purchased from National Center for Clinical Laboratories.